Structural insight into dGTP-dependent activation of tetrameric SAMHD1 deoxynucleoside triphosphate triphosphohydrolase SAMHD1 is a dGTP-activated deoxynucleoside triphosphate triphosphohydrolase (dNTPase) whose dNTPase activity has been linked to HIV/SIV restriction. The mechanism of its dGTP-activated dNTPase function remains unclear. Recent data also indicate that SAMHD1 regulates retrotransposition of LINE-1 elements. Here we report the 1.8-Å crystal structure of homotetrameric SAMHD1 in complex with the allosteric activator and substrate dGTP/dATP. The structure indicates the mechanism of dGTP-dependent tetramer formation, which requires the cooperation of three subunits and two dGTP/dATP molecules at each allosteric site. Allosteric dGTP binding induces conformational changes at the active site, allowing a more stable interaction with the substrate and explaining the dGTP-induced SAMHD1 dNTPase activity. Mutations of dGTP binding residues in the allosteric site affect tetramer formation, dNTPase activity and HIV-1 restriction. dGTP-triggered tetramer formation is also important for SAMHD1-mediated LINE-1 regulation. The structural and functional information provided here should facilitate future investigation of SAMHD1 function, including dNTPase activity, LINE-1 modulation and HIV-1 restriction. SAM domain and HD domain containing protein 1 (SAMHD1) has been linked to the regulation of innate immune responses, and mutations in SAMHD1 have been identified in Aicardi–Goutières syndrome (AGS) patients exhibiting improper immune activation [1] , [2] , [3] . Recently, SAMHD1 has also been shown to function as a potent cellular restriction factor against retroviruses such as HIV and SIV in myeloid cells and resting CD4+ T cells [4] , [5] , [6] , [7] , [8] , [9] , [10] . Virion-associated Vpx protein [11] , [12] , [13] , [14] , [15] , [16] , [17] neutralizes the antiviral activity of SAMHD1 by promoting its proteasome-dependent degradation [5] , [6] . Vpx binds DCAF1 using conserved motifs in helix 1 and helix 3, which in turn recruit other components of the CRL4(DCAF1) E3 ubiquitin ligase [9] , [18] , [19] , [20] , [21] , [22] , [23] to facilitate SAMHD1 ubiquitination and subsequent degradation [4] , [5] , [6] , [18] , [19] , [21] , [22] , [23] . SAMHD1 possesses deoxynucleoside triphosphate triphosphohydrolase (dNTPase) activity [24] , [25] . The dNTPase activity of SAMHD1 is activated by dGTP [24] , [25] and is associated with retroviral restriction in myeloid cells and resting CD4+ T cells as a result of intracellular dNTP depletion [7] , [9] , [26] . However, the mechanism responsible for dGTP-triggered activation of the SAMHD1 dNTPase is not yet clear. The only available crystal structure for SAMHD1 aa 120–626 (SAMHD1c) is a dimer form that lacks the allosteric activator dGTP and substrate dNTP [24] . The crystal structure of the tetramer is particularly desirable, because the formation of SAMHD1 tetramers is critical for its dNTPase activity [27] and may offer useful insight regarding the allosteric activation of SAMHD1 by dGTP. In the current study, we present the crystal structure of homotetrameric SAMHD1 in complex with the allosteric activator and substrate dGTP/dATP at 1.8 Å resolution. The structure reveals the mechanism of dGTP-dependent tetramer formation involving the cooperation of three subunits and two dGTP/dATP molecules at each allosteric site. Allosteric dGTP binding induces conformational changes at the active site, explaining the dGTP-induced SAMHD1 dNTPase activity. Mutations of dGTP binding residues in the allosteric site of SAMHD1 affect tetramer formation, dNTPase activity, HIV-1 restriction and LINE-1 regulation. SAMHD1 tetramer is required for optimal dNTPase activity The SAM domain and its amino-terminal region are not required for tetramer formation or the dNTPase activity of SAMHD1 (refs 27 , 28 ). However, SAMHD1c (120–626) is unable to form tetramers efficiently [24] . It is possible that amino acids preceding residue 120 but downstream of the SAM domain are important for SAMHD1 tetramer formation. Indeed, we have observed that purified SAMHD1 (109–626, SAMHD1c′) readily forms tetramers ( Fig. 1a–c ). On the other hand, we were unable to obtain efficient tetramers with purified SAMHD1c, consistent with previous observations [24] . Purified SAMHD1c′ existed as two major forms in size-exclusion chromatography ( Fig. 1a ). The faster-eluting form (peak 1) had an estimated molecular mass of 280 kDa, consistent with a homotetramer of SAMHD1c′. The slower-eluting form (peak 2) is likely to be monomer SAMHD1c′, although the existence of the dimer could not be ruled out. Both forms predominantly consisted of SAMHD1c′ proteins, as assessed by SDS–polyacrylamide gel electrophoresis (SDS–PAGE) and Coomassie Brilliant Blue staining ( Fig. 1b ). Analytical ultracentrifugation confirmed the existence of the tetramer, as well as monomer forms and a small amount of dimer ( Fig. 1c ). SAMHD1c′ tetramer formation could be induced by dGTP, but not by dATP, dCTP or dTTP ( Fig. 1d ), consistent with the idea that dGTP allosterically regulates SAMHD1 structure and function [24] . We have also observed that formation of the tetramer significantly enhanced the dNTPase activity of SAMHD1 ( Fig. 1e ). Purified SAMHD1c′ resulted in almost complete dGTP hydrolysis after 0.5 h, whereas SAMHD1c produced little hydrolysed substrate after 3 h ( Fig. 1e ). Even at a tenfold higher concentration of SAMHD1c, ~56% of the substrate still remained in the presence of SAMHD1c after 24 h of incubation ( Supplementary Fig. S1 ). Thus, SAMHD1c′ is a much more active dNTPase than is SAMHD1c. 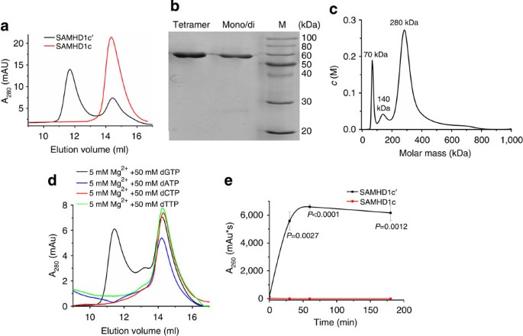Figure 1: Tetramer SAMHD1 is induced by dGTP and possesses a more potent dNTPase activity than the dimer. (a) SAMHD1c′ (SAMHD1 109–626), but not SAMHD1c (SAMHD1 120–626), forms tetramers. Purified recombinant SAMHD1c′ and SAMHD1c proteins were incubated with 50 μM dGTP and separated by size-exclusion chromatography. The elution profiles were monitored by ultraviolet absorbance atA280 nmand compared with known molecular size markers. (b) Both tetramer and monomer peaks contained predominantly SAMHD1c′ proteins, as analysed by SDS–PAGE and Coomassie Brilliant Blue staining. (c) Analytical ultracentrifugation confirmed the existence of the SAMHD1c′ homotetramer. Molecular weights were determined by equilibrium ultracentrifugation at 72,600 g at 16 °C for 4 h in 20 mM Tris–HCl, pH 8.0, with 200 mM NaCl, 5 mM MgCl2, 25 μM dATP and 25 μM dGTP at protein concentrations of 1 mg ml−1. The main peak is centred at 280,000 Da. (d) dGTP, but not dATP, dCTP or dTTP (50 uM), induces the formation of SAMHD1c′ tetramer. (e) SAMHD1c′ has a more potent dNTPase activity than SAMHD1c. Purified recombinant SAMHD1c′ and SAMHD1c proteins were incubated with 1 mM dGTP for the indicated time points at 25 °C. The amount of dG generated at each indicated time point, as described in Methods, is shown here. The s.e. from triplicate samples (n=3) is shown. Student’st-test was performed with Microsoft Excel to generateP-values. Figure 1: Tetramer SAMHD1 is induced by dGTP and possesses a more potent dNTPase activity than the dimer. ( a ) SAMHD1c′ (SAMHD1 109–626), but not SAMHD1c (SAMHD1 120–626), forms tetramers. Purified recombinant SAMHD1c′ and SAMHD1c proteins were incubated with 50 μM dGTP and separated by size-exclusion chromatography. The elution profiles were monitored by ultraviolet absorbance at A 280 nm and compared with known molecular size markers. ( b ) Both tetramer and monomer peaks contained predominantly SAMHD1c′ proteins, as analysed by SDS–PAGE and Coomassie Brilliant Blue staining. ( c ) Analytical ultracentrifugation confirmed the existence of the SAMHD1c′ homotetramer. Molecular weights were determined by equilibrium ultracentrifugation at 72,600 g at 16 °C for 4 h in 20 mM Tris–HCl, pH 8.0, with 200 mM NaCl, 5 mM MgCl 2 , 25 μM dATP and 25 μM dGTP at protein concentrations of 1 mg ml −1 . The main peak is centred at 280,000 Da. ( d ) dGTP, but not dATP, dCTP or dTTP (50 uM), induces the formation of SAMHD1c′ tetramer. ( e ) SAMHD1c′ has a more potent dNTPase activity than SAMHD1c. Purified recombinant SAMHD1c′ and SAMHD1c proteins were incubated with 1 mM dGTP for the indicated time points at 25 °C. The amount of dG generated at each indicated time point, as described in Methods, is shown here. The s.e. from triplicate samples ( n =3) is shown. Student’s t -test was performed with Microsoft Excel to generate P -values. Full size image Tetramer structure of SAMHD1 We have co-crystallized SAMHD1c′ with its dGTP/dATP substrates and solved the structure by the molecular replacement method, using 3U1N (SAMHD1c) as the initial model. Details of data collection and structure refinement are given in Table 1 . The overall structure of SAMHD1 reveals a tetramer, demonstrating tight interactions among four subunits (chains). The asymmetric unit contains a homodimer related by a non-crystallographic twofold axis, and two homodimers are arranged around a crystallographic twofold axis, thus forming a tetrameric assembly with an ~222 symmetry ( Fig. 2 ). We observed 12 dGTP/dATP molecules, 4 Zn 2+ and 4 Mg 2+ per tetramer complex. The interface between chains A and C has not been observed in SAMHD1c ( Fig. 2b ). Table 1 Data collection and refinement statistics. 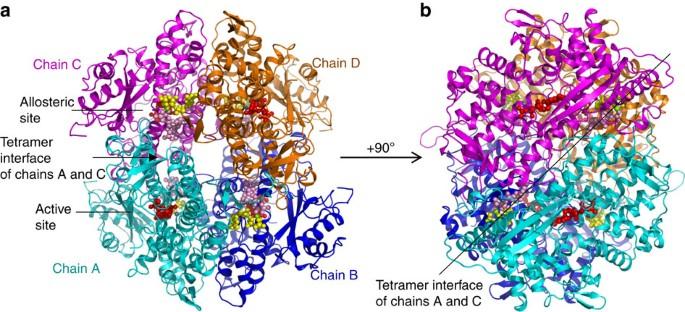Figure 2: Architecture of the SAMHD1 tetramer. (a) A ribbon representation. A substrate (red) and Zn2+(grey) at the active site, two dGTP activators (yellow and pink) and Mg2+(green) at the allosteric site are shown as spheres. The interface between chains A and C is not seen in 3U1N. Chains A and B also exist in 3U1N as a dimer. (b) Rotated around the vertical axis by 90°. The novel symmetric interface between chains A and C is separated by a line. Full size table Figure 2: Architecture of the SAMHD1 tetramer. ( a ) A ribbon representation. A substrate (red) and Zn 2+ (grey) at the active site, two dGTP activators (yellow and pink) and Mg 2+ (green) at the allosteric site are shown as spheres. The interface between chains A and C is not seen in 3U1N. Chains A and B also exist in 3U1N as a dimer. ( b ) Rotated around the vertical axis by 90°. The novel symmetric interface between chains A and C is separated by a line. Full size image Each chain subunit contains major and minor lobes, and a carboxy-terminal region ( Fig. 3a ) with distinct electrostatic potential surface areas ( Supplementary Fig. S2 ). The secondary structure of each chain reveals a mixed α/β dimer ( Supplementary Fig. S3 ). The first two β-strands were not observed in the previous SAMHD1c dimer structure (missing the β1 sequence) [24] . The addition of β1 (115–120) induces the formation of β2 ( Fig. 3a , blue arrow), which is disordered in the SAMHD1c structure. The addition of β1 also appears to be critical for the formation and/or maintenance of the tetramer structure ( Fig. 1 ). The CDK1 phosphorylation site T592, which influences HIV-1 restriction [29] , [30] , and the surrounding amino acids could also be observed for the first time ( Fig. 3a , red arrow). 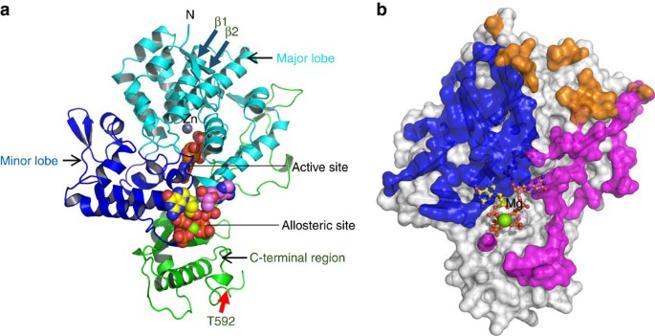Figure 3: Features of a single chain in the SAMHD1 tetramer. (a) A representation of the SAMHD1 monomer with the major lobe, minor lobe and C-terminal region. The first two β-strands in SAMHD1c′ tetramer structure are indicated by a blue arrow. The CDK1 phosphorylation site T592 and the surrounding amino acids are indicated by a red arrow. (b) A surface representation in the same position as ina. The regions at the surface of chain A that are buried by chains B, C and D (shown in blue, purple and orange, respectively). The blue, purple and orange interface areas are ~1,800, 2,100 and 600 Å2, respectively, as calculated by the PDBePISA website. Figure 3: Features of a single chain in the SAMHD1 tetramer. ( a ) A representation of the SAMHD1 monomer with the major lobe, minor lobe and C-terminal region. The first two β-strands in SAMHD1c′ tetramer structure are indicated by a blue arrow. The CDK1 phosphorylation site T592 and the surrounding amino acids are indicated by a red arrow. ( b ) A surface representation in the same position as in a . The regions at the surface of chain A that are buried by chains B, C and D (shown in blue, purple and orange, respectively). The blue, purple and orange interface areas are ~1,800, 2,100 and 600 Å 2 , respectively, as calculated by the PDBePISA website. Full size image The tetramer structure reveals extensive protein–protein interfaces that have not been previously seen ( Fig. 3b ). Each chain (subunit) interacts with all three neighbouring chains. The buried area between chain A and chain B (1,800 Å 2 ) is similar to the dimer structure of SAMHD1c. The buried area between chain A and chain C (2,100 Å 2 ) has not been observed before ( Fig. 3b , purple). Chain A and chain D (600 Å 2 ) also interact ( Fig. 3b , orange), a phenomenon that is not observed in SAMHD1c. The novel interactions between chain A and chain C, as well as between chain A and chain D, are important for dGTP-induced tetramer formation (see below). Allosteric site of SAMHD1 tetramer The dNTPase activity of SAMHD1 is stimulated by dGTP [24] , [25] . dGTP, but not the other dNTPs, is also required for the formation/maintenance of the SAMHD1 tetramer ( Fig. 1 ). A detailed view of the dGTP-binding site provides an explanation for the stabilization of the SAMHD1c′ tetramer by dGTP. Two dGTP molecules or one dGTP and one dATP per allosteric site are extensively coordinated by various amino acids from three separate subunits in the tetramer ( Fig. 4 and Supplementary Fig. S4 ). The addition of amino acids 109–119 of SAMHD1 enhanced tetramer formation ( Fig. 1 ). K116 and N119 from the first β-sheet (green) form H bonds with dGTP molecules ( Fig. 4a ), explaining why SAMHD1c′ could form tetramers. It is interesting to note that only the dGTP-1 molecule was detected at one position in all allosteric sites, whereas one dGTP or one dATP molecule was detected at the other position in the allosteric sites ( Supplementary Fig. S5 ). Specific interactions between R145 and Q142 with the oxygen group of dGTP-1 base provide an explanation for dGTP as the unique activator of SAMHD1. 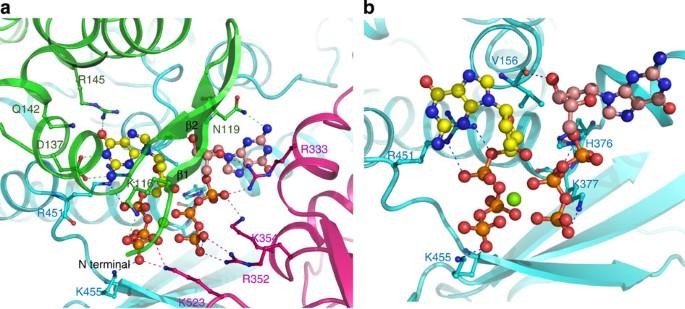Figure 4: Detailed views of the interactions in the allosteric site. (a) Both dGTP molecules are buried in the allosteric site cavity formed by three chains (green, pink and blue). Contributions from all three chains are critical for dGTP binding and allosteric site stability. Interactions contributed by the chains in green and pink are shown. K116 and N119 (from the green chain) located in the first β-sheet (β1) form H bonds with the dGTP molecule. (b) Interactions contributed by the blue chain are shown. Figure 4: Detailed views of the interactions in the allosteric site. ( a ) Both dGTP molecules are buried in the allosteric site cavity formed by three chains (green, pink and blue). Contributions from all three chains are critical for dGTP binding and allosteric site stability. Interactions contributed by the chains in green and pink are shown. K116 and N119 (from the green chain) located in the first β-sheet (β1) form H bonds with the dGTP molecule. ( b ) Interactions contributed by the blue chain are shown. Full size image The details of the interface between chains A and C provided useful information regarding tetramer formation and the allosteric activation of SAMHD1 dNTPase activity. The interface is symmetric between the two chains around the axis ( Fig. 5a , shown in the middle as a line). A helix (A351–V378, shown in cyan and red from two chains) has a key role in the interaction between chains A and C. One side of the helix (D361) from one chain (pink) interacts with the helix (H364 and R372) from another chain (blue). Reciprocal interactions also exist between these two helices ( Fig. 5a ). Two ends of the helix (R352, H376 and K377) bind to the dGTP molecules in the allosteric sites, thus stabilizing the tetramer structure. The other sides (R366 and Y374) of the helices interact with the substrates in the active sites, directly linking changes in the allosteric sites with the substrate binding in the active sites. 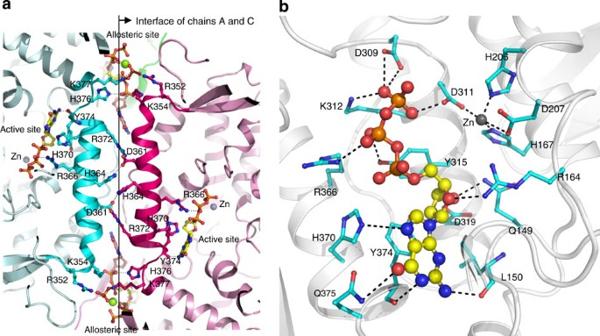Figure 5: A detailed view of the interaction between chains A and C, and substrate interaction in the active site. (a) The symmetric interface between two molecules around the axis (shown in the middle as a line). Helix A351–V378 (shown in blue and purple from different chains) has a key role in this interaction. (b) A close-up view of the active site. The substrate is shown in the ball-and-stick model. The residues shown as blue sticks interact directly with dGTP, and all of them are from one chain. Figure 5: A detailed view of the interaction between chains A and C, and substrate interaction in the active site. ( a ) The symmetric interface between two molecules around the axis (shown in the middle as a line). Helix A351–V378 (shown in blue and purple from different chains) has a key role in this interaction. ( b ) A close-up view of the active site. The substrate is shown in the ball-and-stick model. The residues shown as blue sticks interact directly with dGTP, and all of them are from one chain. Full size image The active site of SAMHD1 tetramer The substrate-binding pocket in the active site is formed by amino acids in the major lobe ( Fig. 5b ). Extensive interactions between the substrate dGTP and surrounding amino acids (including Gln149, Arg164, Lys312, His370 and Tyr374) were observed ( Fig. 5b and Supplementary Fig. S6 ). Substrate dATP in the catalytic site was also observed, consistent with the fact that SAMHD1 can hydrolyse different dNTPs. As in a previous report [24] , the zinc ion is coordinated by the side chains of two histidine (His167 and His206) and two aspartate residues (Asp207 and Asp311). Comparing the dGTP-bound tetramer complexed with substrate to the non-substrate-bound dimer (3U1N) revealed interesting structural differences. Helices (A351–V378) from two neighbouring subunits interact with each other and are critical for tetramer formation. Helices (A351–V378) from two separate subunits are linked by two dGTP molecules at both ends that are part of the allosteric sites. The participation of the first two β-sheets from the third subunit further stabilizes the interaction. In the presence of dGTP molecules, the helix (A351–V378) moves towards the active site (~10°), enabling better substrate binding ( Fig. 6 ). Similarly, amino acids (149–158 and 372–378) in the tetramer also become closer to the active site than those in the 3U1N dimer ( Supplementary Fig. S7 ). Thus, dGTP molecules enhance the tetramer formation and stability that subsequently make the pocket of the active site more suitable for tight substrate interaction in the correct orientation. 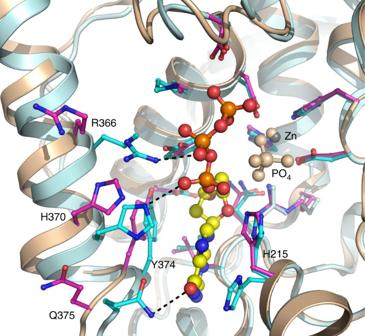Figure 6: A detailed comparison of active sites from our structure and 3U1N. Close-up view of differences in the active sites. The residues in our structure are shown as blue sticks that bind the substrate directly. The corresponding residues in 3U1N are shown as purple sticks. The side chains of R366 and Q375 of 3U1N are oriented in different directions. Figure 6: A detailed comparison of active sites from our structure and 3U1N. Close-up view of differences in the active sites. The residues in our structure are shown as blue sticks that bind the substrate directly. The corresponding residues in 3U1N are shown as purple sticks. The side chains of R366 and Q375 of 3U1N are oriented in different directions. Full size image The catalytic site of the SAMHD1 tetramer structure is significantly different from the catalytic site structure of the reported SAMHD1 dimer (3U1N). 3U1N is shown in wheat colour for comparison ( Fig. 6 ). The α-helix (351–378) is closer to the substrate in the tetramer structure than in the dimer structure ( Fig. 6 ). Arg366 and Gln375 are making direct contact with the substrate in the tetramer, whereas the side chains of these two residues point away from the putative substrate in 3U1N ( Fig. 6 ). Proper alignment of the substrate in the active site is trigged by dGTP binding within the allosteric site, explaining why the tetramer is a more active dNTPase than the dimer. Functional importance of the SAMHD1 tetramer To determine the importance for tetramer formation of dGTP/dATP binding in the allosteric site, we tested several SAMHD1 mutants. These mutations were created to destroy hydrogen bonding with the dGTP/dATP molecules in the allosteric sites of SAMHD1. SAMHD1c′Q142E/R145K, SAMHD1c′R333E/R451E, SAMHD1c′R333E, SAMHD1c′R451E and SAMHD1c′D137A, all had a reduced ability to form tetramers when compared with SAMHD1c′ ( Fig. 7a–f ). The SAMHD1 mutants that are defective for tetramer formation also had reduced dNTPase activity when compared with SAMHD1c′ ( Fig. 7g ). 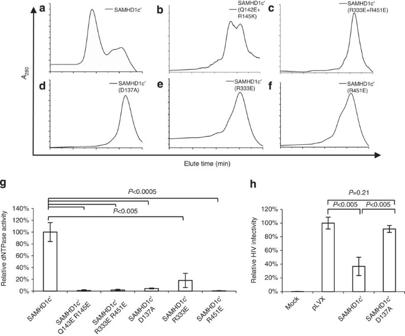Figure 7: Tetramer formation of SAMHD1 is required for dNTPase activity and HIV-1 regulation. (a–f) Mutations of residues involved in dGTP binding in the allosteric site of SAMHD1 affect tetramer formation. Purified recombinant SAMHD1c′ and SAMHD1c′ mutant proteins were incubated with 50 μM dGTP and separated by size-exclusion chromatography. The elution profiles were monitored by ultraviolet absorbance atA280 nmand compared with known molecular size markers. (g) Mutations of residues involved in dGTP binding in the allosteric site of SAMHD1c′ affect dNTPase activity. Purified recombinant SAMHD1c′ and SAMHD1c′ mutant proteins were analysed for dNTPase activity as described in Methods, and the activity of SAMHD1c′ was set to 100%. The s.e. from triplicate samples (n=3) is shown. (h) Tetramer formation is required for SAMHD1-mediated restriction of HIV-1. U937 cells were transduced with pLVX puro-based SAMHD1 expression vectors. Transduced U937 cells were differentiated into macrophages by PMA (phorbol 12-myristate 13-acetate) treatment and infected with HIV-1 EGFP viruses. GFP-positive cells were analysed 2 days after infection by flow cytometry. The experiment was repeated for three times (n=3). The error bars indicated the s.d. of three replicates. Student’st-test was performed with Microsoft Excel to generateP-values. Figure 7: Tetramer formation of SAMHD1 is required for dNTPase activity and HIV-1 regulation. ( a – f ) Mutations of residues involved in dGTP binding in the allosteric site of SAMHD1 affect tetramer formation. Purified recombinant SAMHD1c′ and SAMHD1c′ mutant proteins were incubated with 50 μM dGTP and separated by size-exclusion chromatography. The elution profiles were monitored by ultraviolet absorbance at A 280 nm and compared with known molecular size markers. ( g ) Mutations of residues involved in dGTP binding in the allosteric site of SAMHD1c′ affect dNTPase activity. Purified recombinant SAMHD1c′ and SAMHD1c′ mutant proteins were analysed for dNTPase activity as described in Methods, and the activity of SAMHD1c′ was set to 100%. The s.e. from triplicate samples ( n =3) is shown. ( h ) Tetramer formation is required for SAMHD1-mediated restriction of HIV-1. U937 cells were transduced with pLVX puro-based SAMHD1 expression vectors. Transduced U937 cells were differentiated into macrophages by PMA (phorbol 12-myristate 13-acetate) treatment and infected with HIV-1 EGFP viruses. GFP-positive cells were analysed 2 days after infection by flow cytometry. The experiment was repeated for three times ( n =3). The error bars indicated the s.d. of three replicates. Student’s t -test was performed with Microsoft Excel to generate P -values. Full size image The tetrameric structure of SAMHD1 reported here is significantly different from the published SAMHD1 dimer ( Supplementary Fig. S8 ). The dGTP-induced dNTPase activity is much higher for the tetramer than for the dimer ( Fig. 1 ). The tetramer has also been associated with more potent HIV-1 restriction. We have also evaluated the importance of tetramer SAMHD1 on HIV-1 restriction. SAMHD1c′ restricted HIV-1 infection of differentiated U937 monocytes ( Fig. 7h ). However, SAMHD1c′D137A, which is defective for tetramer formation, had compromised ability to restrict HIV-1 in the same system ( Fig. 7h ). Another functional property of SAMHD1 is its sensitivity to Vpx-mediated degradation [5] , [6] . We next addressed the question of whether tetramer formation is important for Vpx-mediated degradation. Similar to full-length SAMHD1, SIVmac Vpx could induce the degradation of SAMHD1c′, resulting in a reduced intracellular level when compared with that in the absence of Vpx ( Supplementary Fig. S9 ). However, Vpx could not induce the degradation of SAMHD1c ( Supplementary Fig. S9 ). In repeated experiments, SAMHD1c′ could be reduced by ~70% in the presence of Vpx, whereas the SAMHD1c level was not affected by Vpx ( Supplementary Fig. S9 ). We have recently observed that the human SAMHD1 protein is a potent suppressor of LINE-1 activity [31] . To determine whether tetramer formation is also important for LINE-1 inhibition, we compared the functional activity of SAMHD1c′ and SAMHD1c against LINE-1, using a well-established reporter system in HEK293T cells [32] , [33] , [34] . The LINE-1 construct 99 PUR RPS EGFP contains an enhanced green fluorescent protein (EGFP) reporter cassette, interrupted by an intron in the opposite transcriptional orientation and inserted into the 3′-untranslated region of a retrotransposition-competent L1, L1-RP ( Supplementary Fig. S10a ). EGFP is expressed only when the LINE-1 transcript is spliced and reverse-transcribed, its complementary DNA is inserted into the host genome and the EGFP reporter gene is expressed from its own cytomegalovirus promoter. Construct 99 PUR JM111 EGFP (JM111), which contains two missense mutations in ORF1 (ref. 32 ), produces no EGFP signal (that is, it is retrotransposition-defective) and was used as a negative control for retrotransposition ( Supplementary Fig. S10a ). SAMHD1c′ potently inhibited LINE-1 retrotransposition in HEK293T cells ( Supplementary Fig. S10 ). When compared with SAMHD1c′, SAMHD1c had a much lower ability to inhibit LI-RP ( Supplementary Fig. S10 ). The dGTP-binding mutant SAMHD1c′D137A also showed a defect in tetramer formation ( Fig. 7d ). The ability of SAMHD1c′D137A to inhibit LINE-1 retrotransposition was also compromised ( Supplementary Fig. S10 ). It has been reported that a mouse LINE-1 assay system could produce a more efficient retrotransposition event in HEK293T cells [35] . We have compared the anti-LINE-1 function of SAMHD1c′ and SAMHD1c in this established assay system. Again, SAMHD1c′ was much more potent than SAMHD1c against mouse LINE-1 retrotransposition ( Supplementary Fig. S11 ). Thus, formation of the SAMHD1 tetramer is important for efficient human and mouse LINE-1 modulation. SAMHD1 is a dGTP-activated dNTPase. The results presented here provide a structural explanation for the dGTP-triggered dNTPase activity of SAMHD1. dGTP binding in the allosteric site promotes the formation of the SAMHD1 tetramer and the conformational changes in the active site. Consequently, tetramer SAMHD1 is the more active form of dNTPase. We have demonstrated that dGTP-binding residues in the allosteric site of SAMHD1 are important for tetramer formation and dNTPase activity. Although previous work has suggested that the SAMHD1c dimer (aa 120–626) has dNTPase activity [24] , we have determined that SAMHD1c′ (aa 109–626) mainly forms tetramers in the presence of dGTP. Furthermore, tetrameric SAMHD1c′ is at least 50 times more active than the dimer form SAMHD1c in terms of dNTPase activity. We note that SAMHD1c′ maintained many of the biological properties of SAMHD1 (1–626), including dGTP-triggered tetramer formation ( Fig. 1 ), dNTPase activity ( Fig. 1 ), sensitivity to Vpx-mediated degradation ( Supplementary Fig. S9 ) and HIV-1 restriction ( Fig. 7 ). In addition, constructs similar to SAMHD1c′ (containing the SAM domain and its N-terminal deletion) have also been reported to possess HIV restriction function [27] , [28] . Unlike SAMHD1c′, which was sensitive to Vpx-mediated degradation [36] , SAMHD1c was resistant to Vpx-mediated degradation ( Supplementary Fig. S9 ). The addition of amino acids 109–119 was important for the dGTP binding, tetramer formation and dNTPase activity of SAMHD1. SAMHD1 requires dGTP for tetramer formation and activation of dNTPase function. However, unlike Enterococcus faecalis dNTPase EF1143, which binds one dGTP molecule in the allosteric site [37] , the allosteric site of tetramer SAMHD1 binds two dNTP molecules. By using both dGTP and dATP as an activator and a substrate, we have observed that one dGTP (dGTP-1) is invariably detected in the tetramer structure, but the other dGTP (dGTP-2) can be replaced by dATP. Interestingly, the oxygen group of dGTP-1 is coordinated by Q142 and R145, whereas the oxygen group of dGTP-2 does not interact with the surrounding amino acids, explaining why it can be replaced with dATP. Mutations of Q142 and R145 resulted in SAMHD1 mutant molecules that could not form tetramers even in the presence of dGTP. The second dNTP (either dGTP-2 or dATP) in the allosteric site is also apparently important for tetramer formation, as R333 mainly interacted with dGTP-2 or dATP, and the SAMHD1R333E mutant had a reduced ability to form tetramers and also had poor dNTPase activity. Thus, our tetramer SAMHD1 structure and mutagenesis assay have revealed a unique mechanism in which dGTP is required as a stimulator of SAMHD1 tetramer formation and dNTPase activation. The dGTP-induced dNTPase activity was much higher for the tetramer than for the dimer ( Fig. 1 ), and SAMHD1 mutants that were defective for tetramer formation also had reduced dNTPase activity ( Fig. 7 ). These data are consistent with the reported observation that purified tetramer SAMHD1 has much more dNTPase activity than the monomer/dimer [27] . Comparing the structure of dGTP-bound SAMHD1c′ to the non-dGTP-bound SAMHD1c revealed the potential mechanism underlying dGTP-activated dNTPase activity. dGTP binding enhanced the interaction between the helices (A351–V378) from two neighbouring subunits, and this interaction was further strengthened by the first two β-sheets from the third subunit. In the presence of dGTP molecules, the helix (A351–V378) moved towards the active site (~10°), enabling better substrate binding ( Fig. 6 ). Similarly, amino acids (149–158 and 372–378) in the tetramer also moved closer to the active site. Thus, the active site in the tetrameric structure of SAMHD1 is optimized for tight substrate interaction in the correct orientation. The dNTPase activity of SAMHD1 has been linked to HIV-1 restriction [4] , [9] , [24] , and the tetramer form is also required for HIV-1 restriction [27] . We have recently observed that human SAMHD1 is a potent inhibitor of endogenous non-long-terminal repeat retroelements, including LINE-1 (ref. 31 ). The ability to modulate LINE-1 retrotransposition also relies on the tetramer structure of SAMHD1. We have observed that SAMHD1c′ forms tetramers and is a potent inhibitor of both human and mouse LINE-1 retrotransposition. However, SAMHD1c was unable to form tetramers and showed a low level of activity against both human and mouse LINE-1. Furthermore, the SAMHD1c′D137A mutant, which could not form tetramers, also exhibited a compromised ability to inhibit LINE-1. Thus, the biological properties of SAMHD1, such as its dNTPase activity, HIV-1 suppression and regulation of LINE-1 retrotransposition, are functionally linked to the tetramer structure. Examination of the SAMHD1 tetramer also revealed interesting information about amino acid mutations reported in AGS patients. These mutations may alter dGTP binding in the allosteric site, substrate hydrolysis in the catalytic site and protein folding as a result of changes in the hydrophobic core of SAMHD1 ( Supplementary Table S1 and Supplementary Fig. S12 ). Mutations of R145 are detected in AGS patients and would be expected to affect mutant protein binding to dGTP, tetramer formation and dNTPase activity, consistent with our mutagenesis results ( Fig. 7 ). Many of the AGS-related mutations also reduce the LINE-1 regulation activity of mutant SAMHD1 molecules [31] . The crystal structure presented here should facilitate future investigation of SAMHD1’s cellular function and retroviral restriction. Plasmid construction The SAMHD1 gene was retrieved from human blood through reverse transcription followed by PCR amplification, and then subcloned into VR1012 (refs 38 , 39 ; containing a cytomegalovirus promoter/enhancer, intron A, multiple cloning sites and bovine growth hormone polyA signal sequence) with an HA tag at the C terminus. Various site mutations in SAMHD1 and truncation mutants of SAMHD1 were introduced using standard site-directed mutagenesis techniques. All mutant constructs were sequence-confirmed; 99 PUR RPS EGFP and 99 PUR JM111 EGFP LINE-1 retrotransposition reporter constructs have been described [33] . Recombinant protein expression and purification The DNAs encoding residues 1–626, 109–626 and 120–626 of human SAMHD1 were generated by PCR with primers containing Bam HI and Sal I cleavage sites (SAMHD1, 1–626F: 5′-GGATCCGATGCAGCGAGCCGATT-3′; SAMHD1, 109–626F: 5′-GGATCCCAAATCCACGTTGATACAATGAA-3′; SAMHD1, 120–626F: 5′-GGATCCTG GTCTCATCCTCAATTTGAAAAAGATCCTATCCATGGCCAC-3′; SAMHD1R: 5′-GTCGACTCACATTGGGTCATCTT-3′). PCR products were cloned into the pET28a-Plus vector with a His6-tag at the N terminus. The expressed proteins were purified by metal-affinity chromatography on chelation resin and size-exclusion chromatography on a Superdex 200 10/300 GL column [40] . The monomer of SAMHD1 was purified without substrates or ions. To determine the effect of various substrates on the formation of the tetramer, purified recombinant SAMHD1c′ was exchanged into buffer containing 20 mM Tris–HCl (pH 8.0), 200 mM NaCl, 5 mM MgCl 2 and 6 mM β-mercaptoethanol. Various substrates (dGTP, dATP, dTTP and dCTP) were added to a final concentration of 25 μM each. The mixtures were incubated at 4 °C for 2 h and then analysed by size-exclusion chromatography. Analytical ultracentrifugation Sedimentation velocity experiments were performed on a Beckman XL-I analytical ultracentrifuge at 16 °C. Protein samples were diluted with 20 mM Tris–HCl, pH 8.0, with 200 mM NaCl, 5 mM MgCl 2 , 25 μM dATP, 25 μM dGTP and 6 mM β-mercaptoethanol at protein concentrations of 1 mg ml −1 . Data were collected at 72,600 g every 3 min at a wavelength of 280 nm. Interference sedimentation coefficient distributions, c(M), were calculated from the sedimentation velocity data by using SEDFIT. Protein crystallization and X-ray data collection For crystallization, the tetramer of SAMHD1 was concentrated at 5 mg ml −1 with 20 mM Tris–HCl buffer containing 5 mM MgCl 2 , 25 mM dGTP, 25 mM dATP, 0.2 M NaCl and 0.5 mM TCEP (tris-(2-carboxyethyl)phosphine). Crystals were grown at 16 °C using the sitting-drop vapour diffusion method. Crystallization was performed under the conditions provided by the commercially available crystallization screening kits. The crystals belonging to space group C2 were grown in 0.1 M MES (2-(N-morpholino)ethanesulphonic acid, pH 6.5) and 25% w/v polyethylene glycol monomethyl ether 550. Diffraction data were collected at 1w2b beamline of the Institute of High Energy Physics, BL17U beamline of the Shanghai Synchrotron Radiation Facility and BL17A beamline of the Photon Factory (Japan), and processed with HKL2000 (ref. 41 ). The tetramer structure was determined by molecular replacement using the Phaser programme [42] from the CCP4 programme suite [43] . One monomer of 3U1N was used in the initial search models. The structure refinement was carried out with Refmac [44] and Phenix [45] . Model building was carried out using Coot [46] . The qualities of the final structures were evaluated using PROCHECK [47] . The Ramachandran plots showed that >90% of the residues were in the most favourable region. Details of data collection and structure refinement are presented in Table 1 . All figures were prepared using Pymol ( http://www.pymol.org/ ) or Ligplot [48] . dNTPase activity assays dNTPase assays were carried out in a reaction buffer containing 20 mM Tris–HCl, pH 7.8, 50 mM NaCl, 5 mM MgCl 2 , appropriate dNTPs each at 1 mM and 8 μM protein at 25 °C. The reactions were initialized and later terminated by addition of the enzyme and 0.5 M EDTA to a 10-mM final concentration of each. A final volume of 250 μl was used for all reactions. Aliquots collected at various time points were spun through an Amicon Ultra 0.5 ml 10-kDa filter (Millipore) at 12,000 g for 20 min. Deproteinized samples were analysed with an Agilent Technologies 1260 Infinity Series HPLC system (Agilent Technology, Santa Clara, CA) using a 150 × 2.0 mm C18 column (Phenomenex). The column was equilibrated at 40 °C in a 10-mM solution of triethylamine in water, pH 4.95 (buffer A). Injected samples were eluted with a 5-min isocratic phase of buffer A, followed by a methanol gradient over 30 min at a flow rate of 0.2 ml min −1 . The absorbance at 260 nm was used to register eluted compounds in all cases. Antibodies The following antibodies were used to detect protein expression: anti-SAMHD1 from Abcam (catalogue number ab67820, with dilution of 1:500), anti-HA from Invitrogen (catalogue number 715500, 1:250) and anti-FLAG from Sigma (catalogue number F1804, 1:2,000). All antibodies were used according to the manufacturers’ protocols. Cell culture and immunoblotting HEK293T cells were grown in DMEM medium with 10% FBS (Hyclone), GlutaMax and Pen-strep (Invitrogen). DNA transfection was carried out using Lipofectamine 2000 (Invitrogen) according to the manufacturer’s instructions. Vpx-induced SAMHD1 degradation was conducted as previously described [23] . Briefly, the expression vector for wild-type SAMHD1 (75 ng), SAMHD1c′ (125 ng) or SAMHD1c (150 ng) was co-transfected with the empty vector or Vpx expression vector in dose manner (400 or 800 ng) into HEK293T cells. Western blotting was performed after 48 h to detect protein expression for both SAMHD1 and Vpx. SAMHD1 expression was analysed by SDS–PAGE and immunoblotting using SAMHD1-specific antibody from Abcam. Full scans of western blottings are provided in Supplementary Fig. S13 . HIV-1 restriction assays U937 cells were transduced with pLVX puro-based lentiviral vectors expressing SAMHD1 variants. Cells were selected with 1 μg ml −1 puromycin for at least 10 days. Transduced cells were differentiated into macrophages with 30 ng ml −1 phorbol 12-myristate 13-acetate and challenged with HIV-1 NL4–3ΔEnvEGFP plus VSV-G expressing the GFP reporter. Flow cytometry using FACSCalibur was performed 2 days post infection for GFP-positive cells. Gating exclusions were based on background fluorescence of mock-infected U937 cells; 10,000 single-cell events per sample were gated and analysed using CellQuest Pro (version 5.2). LINE-1 retrotransposition assay The human L1 plasmids 99 PUR L1-RP EGFP (L1) and 99 PUR JM111 EGFP (JM111, as a negative control) have been previously described [33] . In brief, LINE-1 plasmid was transfected into HEK293T cells at 2 μg per well in 12-well plates, together with the empty vector VR1012 or one of the test plasmids. The cells were selected by the addition of puromycin (final concentration, 5 μg ml −1 ) at 48 h post transfection. GFP-positive cells were examined 48 h later by flow cytometry using FACSCalibur. Gating exclusions were based on the background fluorescence of the plasmid 99 PUR JM111 EGFP, a LINE-1 construct containing two point mutations in ORF1 that completely abolish retrotransposition; 10,000 single-cell events per sample were gated and analysed using CellQuest Pro (version 5.2). Accession codes: Coordinates and structure factors have been deposited in the RCSB protein data bank under accession code 4MZ7 . How to cite this article: Zhu, C. et al. Structural insight into dGTP-dependent activation of tetrameric SAMHD1 deoxynucleoside triphosphate triphosphohydrolase. Nat. Commun. 4:2722 doi: 10.1038/ncomms3722 (2013).